A cobalt complex redox shuttle for dye-sensitized solar cells with high open-circuit potentials Dye-sensitized solar cells are a promising alternative to traditional inorganic semiconductor-based solar cells. Here we report an open-circuit voltage of over 1,000 mV in mesoscopic dye-sensitized solar cells incorporating a molecularly engineered cobalt complex as redox mediator. Cobalt complexes have negligible absorption in the visible region of the solar spectrum, and their redox properties can be tuned in a controlled fashion by selecting suitable donor/acceptor substituents on the ligand. This approach offers an attractive alternate to the traditional I 3 − /I − redox shuttle used in dye-sensitized solar cells. A cobalt complex using tridendate ligands [Co(bpy-pz) 2 ] 3+/2+ (PF 6 ) 3/2 as redox mediator in combination with a cyclopentadithiophene-bridged donor-acceptor dye (Y123), adsorbed on TiO 2 , yielded a power conversion efficiency of over 10% at 100 mW cm −2 . This result indicates that the molecularly engineered cobalt redox shuttle is a legitimate alternative to the commonly used I 3 − /I − redox shuttle. The dye-sensitized solar cell (DSC) is a promising alternative to traditional inorganic semiconductor-based solar cells because of favourable ecological and economical features. Sun light is absorbed by a dye monolayer located at the junction between a nanostructured electron transporting (n-type) and hole-transporting (p-type) phase. The former is a wide bandgap semiconductor oxide (typically TiO 2 , anatase), and the latter is typically the triiodide/iodide (I 3 − /I − ) redox electrolyte [1] , [2] . On photo-excitation, the dye injects an electron into the n-type material and the hole is captured by the electrolyte. The electrons then travel through the nanostructure to be collected as current at the external contact [3] , while the holes are transported to the cathode by the redox shuttle. The main drawback of the commonly used triiodide/iodide redox (I 3 − /I − ) system is a large mismatch between its oxidation potential ( E 0 (I 3 − /I − )=0.35 V versus the normal hydrogen electrode (NHE)) and the dye oxidation potential ( E 0 (S + /S)=~1.0 V versus NHE), which limits the open circuit voltage ( V oc ) to 0.7–0.8 V (ref. 4 ). The large expenditure needed for efficient dye regeneration is due to the complex regeneration kinetics with the I 3 − /I − redox couple involving formation of intermediates that is, the I 2 − radical [5] , [6] . Additionally, this redox couple is very corrosive towards metals such as Ag, Au and Cu, so excluding the use of such materials as current collectors in DSC modules requiring long-term stability. Therefore, the development of non-corrosive redox mediators, with reduced mismatch between the oxidation potential of the dye and the redox couple, is paramount to enhancing open circuit potential. Previous studies to replace the I 3 − /I − redox system by cobalt polypyridine complexes have drawn attention because of their low visible light absorption, the higher redox potential and the reduced corrosiveness towards metallic conductors offered by these redox couples [7] , [8] . However, the overall efficiency obtained with these cobalt electrolytes was inferior compared with the I 3 − /I − couple, especially under full sunlight. This has been attributed to slow mass transport [8] , [9] and faster back reaction of photo-injected electrons with the oxidized redox species [10] coupled with the slow regeneration of the Co(II) species at the cathode [11] . Recently, cobalt redox shuttles have attracted renewed attention after Feldt et al . [12] increased the power conversion efficiency (PCE) to 6.7% by employing a newly designed D-π-A organic sensitizer, coded D35, in conjunction with the cobalt (III/II) tris-bipyridyl complex, [Co(III)(bpy) 3 ](PF 6 ) 3 /[Co(II)(bpy) 3 ](PF 6 ) 2 couple [13] , [14] , [15] . Most recently, S. M. Feldt et al . have achieved over 1,000 mV with cells based on cobalt phenanthroline redox shuttles but the power conversion efficiencies were below 3.6% (ref. 16 ). As cobalt is a first row transition metal, dissociation and exchange of ligands may occur rapidly in the case of Co(II). Tridentate ligands are expected to improve significantly the stability of the cobalt complex compared with bidentate ligands. Another advantage of tridentate ligands over bidentate ligands is the absence of isomers. Thus, in the case of dissymmetric bidentate ligands, useful for fine tuning of the redox properties, facial and meridional isomers coexist. One particular attractive feature of cobalt complexes is the facile tuning of their redox potential, which can be adjusted to match the oxidation potential of the sensitizer minimizing energy loss in the dye regeneration step. We report a redox relay that can generate a high potential and, thus, highly efficient DSCs with [Co(III/II)(bpy-pz) 2 ](PF 6 ) 3/2 (denoted hereafter as [Co(bpy-pz) 2 ] 3+/2+ ) [bpy-pz=6-(1 H -pyrazol-1-yl)-2,2′-bipyridine]). The tridentate cobalt [Co(bpy-pz) 2 ] 3+/2+ (PF 6 ) 3/2 complex, used as a redox mediator, achieved an unprecedented output voltage exceeding 1,000 mV owing to its high oxidation potential of 0.86 V versus NHE. The designed complex [Co(bpy-pz) 2 ] 3+/2+ ( Fig. 1 ), whose redox potential is offset by only 230 mV from that of the 3-{6-{4-[bis(2′,4′-dihexyloxybiphenyl-4-yl)amino-]phenyl}-4,4-dihexyl-cyclopenta-[2,1-b:3,4-b]dithiphene-2-yl}-2-cyanoacrylic acid ( Y123 ) dye gave a PCE of over 10%, under different solar intensities from 10 to 100 mW cm −2 . 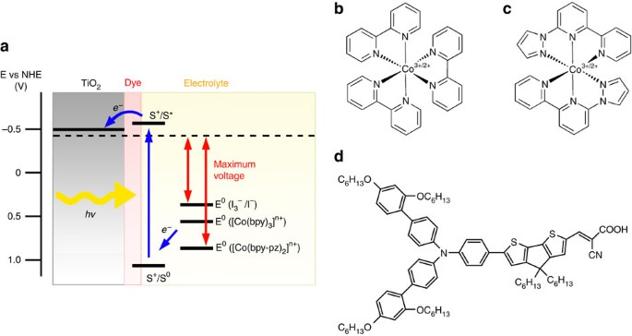Figure 1: Schematic energy diagram for dye-sensitized solar cell. (a) TiO2sensitized with Y123 dye. (b) Molecular structures of tris bipyridine cobalt complex. (c) Molecular structures of bis bipyridine-pyrazole cobalt complex. (d) Molecular structures of Y123 dye. Figure 1: Schematic energy diagram for dye-sensitized solar cell. ( a ) TiO 2 sensitized with Y123 dye. ( b ) Molecular structures of tris bipyridine cobalt complex. ( c ) Molecular structures of bis bipyridine-pyrazole cobalt complex. ( d ) Molecular structures of Y123 dye. Full size image Electrochemical data The standard redox potential of the [Co(bpy-pz) 2 ] 3+/2+ couple was determined as 0.22 V versus ferrocenium/ferrocene (Fc + /Fc) (0.86 V versus NHE using E 0 (Fc + /Fc)=0.64 V versus NHE) by cyclic voltammetry ( Supplementary Fig. S1 ). The higher oxidation potential compared with [Co(bpy) 3 ] 3+/2+ is attributed to the presence of pyrazoles, which stabilize the highest occupied molecular orbital (HOMO) of the complex more than the bipyridine ligand. For the Co(bpy-pz) 2 ] 3+/2+ containing 0.22 M of Co(II) and 0.05 M Co(III), the calculated redox potential is 0.82 V versus NHE whereas, for the I 3 − /I − -based electrolyte, the value is 0.37 V versus NHE. The absorption spectra of the oxidized species [Co(bpy-pz) 2 ] 3+ show maxima: λ max ( ɛ )=265 (28,300), 320 nm (24,400), and, for reduced species [Co(bpy-pz) 2 ] 2+ λ max ( ɛ )=240 (35,500), 276 nm (20,500) ( Supplementary Fig. S2 ). Strong π accepting nature of pyrazoles increased HOMO–LUMO (lowest unoccupied molecular orbital) gap, hence reduced its absorption in the visible spectrum compared with [Co(bpy) 3 ] 3+/2+ systems. It is worthy to note that triiodide has a molar extinction coefficient of 25,500 at 360 nm [17] . The additional photocurrent generated by the sensitizer in the blue part of the spectrum is expected with the use of the cobalt electrolyte system compared with the (I 3 − /I − ) due to the lower extinction coefficient of the cobalt complexes. Dye sensitized solar cell The redox reactions of dye sensitized solar cells (DSCs) under illumination will be briefly presented. Details can be found elsewhere [18] , [19] , [20] . The photo-excitation of the adsorbed sensitizer on nanocrystalline semiconductor (equation (1)) leads to injection of electrons into the conduction band of the semiconductor (equation (2)). The oxidized dye is subsequently reduced by electron donation from an electrolyte containing the redox system (equation (3)). The injected electron flows through the semiconductor network to arrive at the back contact of the anode and then through the external load to the counter electrode. At the counter electrode, reduction of oxidized component of the redox couple in turn regenerates the reduced form (equation (4)), which completes the circuit. With a closed external circuit and under illumination, the device then constitutes a photovoltaic regenerative energy conversion system. However, there are undesirable loss reactions, such as the injected electrons may recombine either with the oxidized sensitizer (equation (5)) or with the oxidized form of the redox couple at the TiO 2 surface (equation (6)), resulting in a loss of cell efficiency. Charge transfer dynamics To gain insight into dye regeneration rate, time-resolved nanosecond laser transient absorbance measurements were performed on both the cobalt and the I 3 − /I − redox systems. The dye regeneration yield, η r is defined by equation (7): where k r is the first-order rate constant of the dye regeneration (equation (3)) occurring in the presence of a redox couple (R + /R). And k b is the rate constant of the recombination reaction (equation (5)) that takes place between the oxidized state of the dye (S + ) and electrons injected into the conduction band following the primary ultrafast photoinduced charge separation process (equations (1) and (2)). The dynamics of the oxidized state of the dye after its initial generation was monitored by measuring transient changes of its optical absorption at the wavelength λ =715 nm. In the absence of a redox mediator, that is, in pure acetonitrile solvent, the decay of the absorption signal recorded at 715 nm reflects the dynamics of the recombination of injected electrons with S + . 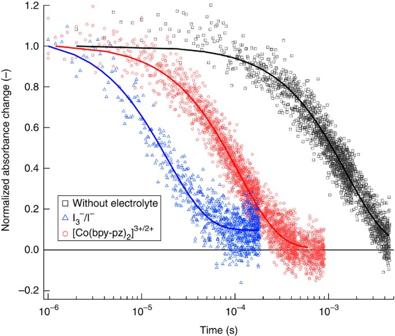Figure 2: Transient absorbance decay kinetics of oxidized dye. The curves show transient absorbance of the oxidized state of the Y123 dye adsorbed on a TiO2nanocrystalline film in pure acetonitrile (black squares), in presence of the [Co(bpy-pz)2]3+/2+-based electrolyte (red circles), and the I3−/I−redox system (blue triangles). In Figure 2 , the black curve shows that the transient absorbance of the oxidized state of the Y123 dye decays with a typical half-reaction time t 1/2 =1.1 ms. Data fitted by a single exponential yielded a rate constant of k b =6.4×10 2 s −1 . In the presence of the redox couple, the decay of the oxidized dye signal was significantly accelerated and the half-reaction time decreased to t 1/2 =80 μs for [Co(bpy-pz) 2 ] 3+/2+ and to 16 μs for I 3 − /I − . The rate constants extracted by fitting with a single exponential are k r =9.1×10 3 s −1 and 5.3×10 4 s −1 for the regeneration of the dye by [Co(bpy-pz) 2 ] 3+/2+ and I 3 − /I − redox systems, respectively [9] . Despite the dissimilar rate constants in the cobalt and the I 3 − /I − system, k r remains much larger than k b indicating that electron recombination with the oxidized dye is indeed intercepted efficiently by the mediator, corresponding to a dye regeneration yield of η r =~0.93 by the [Co(bpy-pz) 2 ] 3+/2+ redox system, whereas the dye regeneration yield by I 3 − /I − is η r >0.98. This efficient dye regeneration yield observed with the [Co(bpy-pz) 2 ] 3+/2+ redox system is particularly noteworthy as the difference in the oxidation potential between the dye and the redox couple is only 230 mV. Larger energy expenditure is usually required for the effective regeneration of the dye [6] , [16] , [21] , [22] . Figure 2: Transient absorbance decay kinetics of oxidized dye. The curves show transient absorbance of the oxidized state of the Y123 dye adsorbed on a TiO 2 nanocrystalline film in pure acetonitrile (black squares), in presence of the [Co(bpy-pz) 2 ] 3+/2+ -based electrolyte (red circles), and the I 3 − /I − redox system (blue triangles). Full size image Photovoltaic data Table 1 summarizes the photocurrent-voltage characteristics of the DSCs employing a 5.6-μm thin transparent nanoporous TiO 2 (anatase) film, the Y123 sensitizer, and the redox electrolytes under simulated sunlight at various intensities: 9.5, 51 and 100 mW cm −2 . The [Co(bpy-pz) 2 ] 3+/2+ redox system gave a photocurrent density of ( J sc ) 12.54 mA cm −2 , an open-circuit potentials ( V oc ) of 1,020 mV and a fill factor ( FF ) of 0.69, yielding a PCE ( η ) of 8.87%, as derived from equation (8): where J sc is the short circuit current density, V oc is the open circuit voltage, FF is the fill factor, and I 0 is the intensity of the simulated sunlight impinging on the solar cell. All averaged J – V characterizations are summarized in Supplementary Table S1 . Under similar conditions, the I − /I 3 − system resulted in J sc =13.01 mA cm −2 , V oc =754 mV, and FF =0.67, yielding a PCE of 6.57%. The V oc of 1,018 mV based on the [Co(bpy-pz) 2 ] 3+/2+ is 264 mV higher than that of the I 3 − /I − system ( Fig. 3a ), which results in an overall PCE increase of 35% over the I 3 − /I − system. Additionally, at lower light intensities, that is, 51 and 9.5 mW cm −2 , the PCE values of 9.3–9.4% were measured that are remarkably high for DSCs with the 5.6-μm thin TiO 2 films used in this study. Table 1 J – V characterization of the DSCs employing 5.6-μm thin thick TiO 2 films. 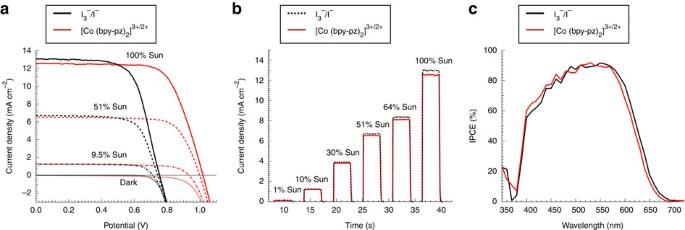Figure 3: Photovoltaic characteristics using cobalt and iodide redox systems. (a) Comparison ofJ–Vcurve for the [Co(bpy-pz)2]3+/2+(red lines) and I3−/I−(black lines). (b) Photo-current dynamics as a function of light intensity for the [Co(bpy-pz)2]3+/2+(red lines) and I3−/I−(black lines). (c) Comparison of IPCE spectra using TiO2film thickness is 5.6 μm and [Co(bpy-pz)2]3+/2+(red lines) and I3−/I−(black lines) redox systems. Full size table Figure 3: Photovoltaic characteristics using cobalt and iodide redox systems. ( a ) Comparison of J – V curve for the [Co(bpy-pz) 2 ] 3+/2+ (red lines) and I 3 − /I − (black lines). ( b ) Photo-current dynamics as a function of light intensity for the [Co(bpy-pz) 2 ] 3+/2+ (red lines) and I 3 − /I − (black lines). ( c ) Comparison of IPCE spectra using TiO 2 film thickness is 5.6 μm and [Co(bpy-pz) 2 ] 3+/2+ (red lines) and I 3 − /I − (black lines) redox systems. Full size image Figure 3b shows the photocurrent dynamics as a function of incident light intensity. The previously reported diffusion problem [8] regarded as a drawback and associated with remarkable loss in photocurrent at full solar intensity was not observed with the [Co(bpy-pz) 2 ] 3+/2+ system. Figure 3c exhibit the incident photon-to-current conversion efficiency (IPCE) spectra of both redox systems showing high values, that is, 70–90% in the 440 and 620 nm wavelength range. Regarding the iodine-based electrolyte, the cobalt [Co(bpy-pz) 2 ] 3+/2+ system exhibited an enhanced photocurrent response in the spectral range from 390 to 480 nm, which is ascribed to the lower molar absorption coefficients of the cobalt [Co(bpy-pz) 2 ] 3+/2+ in the blue spectral region compared with I 3 − /I − . To further investigate our devices, we took a closer look at the dark current. The dark current is generally dominated by the recombination through nanocrystalline TiO 2 particles after TiCl 4 treatment [23] or the fluorine-doped transparent tin oxide (FTO) exposed to the electrolyte. The DSC with the I 3 − /I − redox system shows a lower dark current near 0 V than the cobalt redox systems, which indicates a higher shunt resistance—in other words, a better blocking of the leakage current at the FTO substrate ( Supplementary Fig. S3 ) [11] . The steep rise of the dark current at higher forward bias is dominated by the reaction of electrons with the oxidized redox species over the mesoporous TiO 2 . For the I 3 − /I − -based DSC, it rises at a lower forward bias potential compared with the cobalt redox electrolytes. This is attributed to the difference of the redox potentials, but a conduction band edge shift could also produce such a result. Electrochemical impedance spectroscopy To clarify the origin of our observation, we performed electrochemical impedance spectroscopy (EIS) measurements. 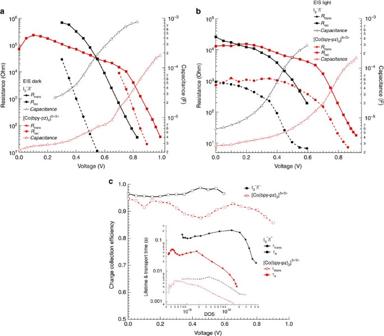Figure 4: EIS results of I3−/I−and [Co(bpy-pz)2]3+/2+system-based DSCs. Transport resistance (Rtrans) (dashed lines), recombination resistance (Rrec) (solid lines), and chemical capacitance (dotted lines) of the [Co(bpy-pz)2]3+/2+(red lines and markers) and I3−/I−(black lines and markers) system-based DSCs (a) in the dark and (b) at 1 sun by light-emitting diode. (c) Charge collection efficiency of I3−/I−(black solid line with open squares) and [Co(bpy-pz)2]3+/2+(red dashed line with closed circles)-based DSCs as function of applied potential. Inset shows the electron lifetime and the transport time for [Co(bpy-pz)2]3+/2+and the I3−/I−plotted against DOS. Figure 4a shows the recombination and the transport resistance as well as the chemical capacitance for the cells based on [Co(bpy-pz) 2 ] 3+/2+ and I 3 − /I − redox electrolyte in the dark. As implied by the dark current near 0 V, the recombination resistance is lower for the [Co(bpy-pz) 2 ] 3+/2+ than the I 3 − /I − redox electrolyte. The chemical capacitance is shifted by ~430 mV, which is due to the differences of the two redox potentials associated with a higher recombination for the cobalt redox system and a small shift in the conduction band (E cb ) of the TiO 2 . Figure 4: EIS results of I 3 − /I − and [Co(bpy-pz) 2 ] 3+/2+ system-based DSCs. Transport resistance ( R trans ) (dashed lines), recombination resistance ( R rec ) (solid lines), and chemical capacitance (dotted lines) of the [Co(bpy-pz) 2 ] 3+/2+ (red lines and markers) and I 3 − /I − (black lines and markers) system-based DSCs ( a ) in the dark and ( b ) at 1 sun by light-emitting diode. ( c ) Charge collection efficiency of I 3 − /I − (black solid line with open squares) and [Co(bpy-pz) 2 ] 3+/2+ (red dashed line with closed circles)-based DSCs as function of applied potential. Inset shows the electron lifetime and the transport time for [Co(bpy-pz) 2 ] 3+/2+ and the I 3 − /I − plotted against DOS. Full size image In Fig. 4b the characteristic parameters of the EIS analysis of the devices under illumination (at 1 sun by a light-emitting diode) are presented and compared. It is noted that the transport and the recombination resistance drop drastically because of the increased charge carriers injected by the dye into the conduction band of TiO 2 ( Supplementary Fig. S4a,b ). The chemical capacitance under illumination is shifted by ~400 mV. Therefore, the density of states (DOS) between two electrolyte systems under illumination, as calculated from the capacitance of the EIS, shows a shift of ~400 mV as shown in Supplementary Figure S4c . Similar to the case of dark EIS, this is also slightly less than the expected 450 mV gain. The electron lifetime and the transport time under illumination are plotted against the DOS (inset in Fig. 4c ; the plot against potential can be found in Supplementary Fig. S4d ). The electron lifetime observed for the [Co(bpy-pz) 2 ] 3+/2+ system is several times shorter than for the I 3 − /I − electrolyte whereas the transport time is comparable. The photovoltaic performance is evidently reflected by the charge collection efficiency derived from η CC =(1+ R trans /R rec ) −1 . The system with the highest η CC is the I 3 − /I − system showing over 95% followed by the [Co(bpy-pz) 2 ] 3+/2+ exhibiting, nevertheless, over 90% ( Fig. 4c ) charge collection efficiency although the recombination is faster. Effect of TiO 2 film thickness on photovoltaic properties To fully characterize the DSC performance with the [Co(bpy-pz) 2 ] 3+/2+ system, the transparent TiO 2 film thickness was varied between 2.8 and 5.6 μm onto which a 5-μm scattering layer was deposited ( Table 2 ; all averaged J – V characterization are summarized in Supplementary Table S2 ). The 2.8-μm transparent layer gave a J sc of 10.80 mA cm −2 , a V oc of 1,031 mV and a FF of 0.68, corresponding to a PCE of 7.52% at full sun, 100 mW cm −1 . The light harvesting efficiency ( LHE ), defined as where ɛ is the molar extinction coefficient of the dye, Γ is the dye molar concentration per projected surface area of the film, and A is the absorbance of the dye-sensitized film (equal to the product of ɛ and Γ) [24] is estimated to be already over 98% at maximum with the 2.8 μm TiO 2 film, which indicates the impact of high molar extinction coefficient dyes. So the photocurrent of 10.80 mA cm −2 was decreased only by 16% when decreasing the TiO 2 film thickness by 50%. At low intensities, 51 and 9.5 mW cm −2 , the devices exhibited dramatically high V oc , 1,013 and 960 mV leading to a PCE of 8.21% and 8.51%, respectively. The introduction of optical elements, that is, layers composed of large particles [25] , [26] , [27] , [28] enhanced the photocurrent owing to incident light scattering towards nanocrystalline mesoporous TiO 2 film. A dye-sensitized solar cell incorporating a 5-μm thick scattering layer on 5.6-μm transparent layer exhibited an enhanced photocurrent of 13.45 mA cm −2 , which is an increase of 7% while retaining V oc and FF when compared with the DSC with 5.6-μm transparent layer. The respective PCE were 9.52, 10.29 and 9.93% at 100, 51 and 9.5 mW cm −2 (see J – V curves in Fig. 5a ). 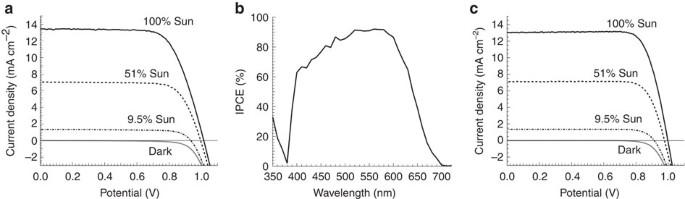Figure 5: Photovoltaic characteristics of DSC based on [Co(bpy-pz)2]3+/2+system. (a)J–Vcharacterization and (b) IPCE of the DSC employing the double-layered TiO2(5.6+5 μm) and Pt counter electrode. (c)J–Vcharacterization of the DSC employing the double-layered TiO2(4.0+4.5 μm) and the PProDOT cathode instead of Pt. Figure 5b shows the IPCE of the cell based on the [Co(bpy-pz) 2 ] 3+/2+ system with a TiO 2 double layer. The IPCE spectrum exhibits very high values, that is, 70–90% between excitation wavelengths of 430 and 620 nm. Assuming a 10% optical loss in the conducting glass, the internal quantum efficiency ranged from 80–100% (ref. 29 ). These overall PCEs with the dramatically high V oc s, is, to the best of our knowledge, an unprecedented result. Given the high V oc , this new cobalt redox relay-based DSC will be also very attractive for use as photovoltaic devices in water cleavage, as the required photovoltage can be reached by merely two cells connected in series to a water electrolyzer, or with just one cell in tandem with a water oxidizing photoanode [30] . A device kept at ambient conditions showed no loss in the conversion efficiency after 1 month, which is a promising result. Further work on stability of this new redox system is ongoing. Table 2 J – V characterization of the DSCs. Full size table Figure 5: Photovoltaic characteristics of DSC based on [Co(bpy-pz) 2 ] 3+/2+ system. ( a ) J – V characterization and ( b ) IPCE of the DSC employing the double-layered TiO 2 (5.6+5 μm) and Pt counter electrode. ( c ) J – V characterization of the DSC employing the double-layered TiO 2 (4.0+4.5 μm) and the PProDOT cathode instead of Pt. Full size image Platinum-free counter electrode A comparatively high charge-transfer resistance, R CT , at the Pt counter electrode with the cobalt redox system was observed despite the promising PCE. To further reduce the R CT , a high surface area-cathode material (that is, nanoporous poly(3,4-propylenedioxythiophene) (PProDOT) [31] layers) was exploited to replace the Pt. With the incorporation of the PProDOT as cathode material, the FF was strongly improved owing to a lower R CT ( Supplementary Table S3 ) and thus the PCE increased to 10.08% at 1 sun illumination ( Table 2 ; Fig. 5c ). The PProDOT layer showed a drastically lower R CT , 2.5 ohms in comparison to the 50 ohms of the counter electrodes made with Pt. It is noted that the R CT of I 3 − /I − system is ~0.8 ohms with Pt counter electrode. The lower V oc , which is plausibly ascribed to the downward shift of the TiO 2 band edge [31] , was compensated by a higher fill factor. Our ongoing study concentrates to develop and analyse diverse alternative cathode materials. We have synthesized novel cobalt (III) and (II) complexes based on 6-(1 H -pyrazol-1-yl)-2,2′-bipyridine tridentate ligand, and used them as a redox couple in mesoscopic dye-sensitized solar cells in conjunction with a high molar extinction coefficient organic donor-π-acceptor dye. Under the 1 sun condition, a very high open-circuit voltage, ~1,000 mV, along with a short circuit current of 13.06 mA/cm 2 , and FF , 0.77 were obtained, resulting in a PCE of above 10%. The high open-circuit voltage was obtained by stabilizing the HOMO level of the cobalt (II) complex to minimize the mismatch between the redox couple and the sensitizer HOMO level to just 230 mV. This resulted in higher PCE compared with the iodide/triiodide redox couple. Also, we found that the conventional Pt catalyst coated counter electrode is not optimum with the newly developed cobalt redox mediators; therefore, to overcome this issue, a series of polythiophene family members were exploited as a cathode material. PProDOT-based counter electrode in DSCs show optimum results owing to their ultrahigh surface area morphology and without the possibility of forming any passivation layer at electrolytes–electrode interface. These promising results not only confirm that the molecularly engineered cobalt redox shuttle is a legitimate alternative to the commonly used I 3 − /I − redox shuttle but also assures improved performance with low-cost materials as a cathode. Future work will focus on further improvements of this potential new redox system, and to increase the recombination resistance. As a possibility, the recombination process could be retarded by depositing a conformal insulating oxide blocking layer on the surface of the TiO 2 films by atomic layer deposition [32] , [33] . We believe that the dye-sensitized solar cell described here is straightforward, which carries the promise of truly inexpensive and environment-friendly solar power. Materials synthesis The synthetic details of 3-{6-{4-[bis(2,4-dihexyloxybiphenyl-4-yl)amino-]phenyl}-4,4-dihexyl-cyclopenta-[2,1-b:3,4-b2]dithiphene-2-yl}-2-cyanoacrylic acid, coded Y123, were described in our previous study [14] . The ligand bpy-pz has been prepared in a similar manner to ligands reported previously [34] , [35] . Spectroscopic analysis gave similar results to that reported in literature [36] . The preparation details of PProDOT-coated FTO as counter electrode has been described in our previous study [31] . In this study, ~160-nm thick PProDOT on FTO was prepared and used as the cathode. [Co(bpy-pz) 2 ](PF 6 ) 2 91 mg (0.382 mmol, excess) of CoCl 2 ·6H 2 O were dissolved in 25 ml of water while, in another flask, 93 mg (0.418 mmol) of bipyridine-pyrazole ligand was dissolved in 25 ml of acetone. The solutions were combined and heated to 55 °C for 2 h. Then, 400 mg of NH 4 PF 6 dissolved in 100 ml of water were added to the mixture. The mixture was stored overnight at 3 °C to aid precipitation. Then, the product was collected on a sintered glass frit and dried in vacuo . The pure product was obtained as an orange solid. Yield: 95 mg (0.12 mmol, 57%). 1 H nuclear magnetic resonance (NMR) (400 MHz, acetone-D6); δ 112.95 (s, 2H, ArH), 91.83 (s, 2H, ArH), 89.23 (s, 2H, ArH), 75.68 (s, 2H, ArH), 69.31 (s, 2H, ArH), 66.22 (s, 2H, ArH), 43.00 (s, 2H, ArH), 40.74 (s, 2H, ArH), 19.01 (s, 2H, ArH), 13.61 (s, 2H, ArH) p.p.m. HRMS (ESI-TOF) m/z (%): calculated for C 26 H 20 CoN 8 PF 6 648.0785; found 648.0805 (17) [(M–PF 6 ) + ]; calculated for C 26 H 20 CoN 8 : 251.5571; found 251.5565 (100) [(M –2PF 6 ) 2+ ]. [Co(bpy-pz) 2 ](PF 6 ) 3 530 mg (2.22 mmol, excess) of CoCl 2 ·6H 2 O was dissolved in 25 ml of water, while, in another flask, 550 mg (2.47 mmol) of the bipyridine-pyrazole ligand was dissolved in 15 ml of acetonitrile. The solutions were combined and H 2 O 2 (4 ml, 30%) and HCl (4 ml, 37%) were added to oxidize the cobalt (II). The mixture was heated to 50 °C for 3 h. A small aliquot (1 ml) was taken out and the product precipitated by adding aq. KPF 6 solution. The solid was collected, dried and analysed by NMR. The solid was collected on a glass-frit, washed with water and Et 2 O and dried in vacuo to obtain the pure product as orange solid. Yield: 355 mg (0.38 mmol, 31%). 1 H NMR (400 MHz, acetone-D6): δ 9.42 (dd, 3 J HH =3.2 Hz, 4 J HH =0.4 Hz, 1H, ArH), 9.35 (t, 3 J HH =8.2 Hz, 1H, ArH), 9.27 (dd, 3 J HH =8.0 Hz, 4 J HH =0.8 Hz, 1H, ArH), 9.01 (dd, 3 J HH =8.3 Hz, 4 J HH =0.8 Hz, 1H, ArH), 8.99 (ddd, 3 J HH =8.0 Hz, 4 J HH =1.4 Hz, 4 J HH =0.4 Hz, 1H, ArH), 8.46 (td, 3 J HH =7.8 Hz, 4 J HH =1.3 Hz, 1H, ArH), 7.93 (br d 3 J HH =5.9 Hz, 1H, ArH), 7.84 (dd, 4 J HH =2.4 Hz, 4 J HH =0.4 Hz, 1H, ArH), 6.87–6.86 (m, 1H, ArH) p.p.m. 19 F NMR (188 MHz, acetone-D): δ −72.3 (d, 1 J PF =707 Hz, PF 6 ) p.p.m. HRMS (ESI-TOF) m/z (%): calculated for C 26 H 20 CoN 8 P 2 F 12 793.0427; found 793.0436 (35) [(M–PF 6 ) + ]; calculated for C 26 H 20 CoN 8 PF 6 648.0785; found 648.0869 (4) [(M–2PF 6 ) + ]; calculated for C 26 H 20 CoN 8 : 251.5571; found 251.5524 (100) [(M –3PF 6 ) 2+ ]. Solar cell fabrication and characterization The nanocrystalline TiO 2 pastes were prepared using a previously reported procedure [23] . The TiO 2 transparent electrodes were prepared by screen printing onto fluorine-doped tin oxide (FTO, Solar 4 mm thickness, 10 ohms per sq, Nippon Sheet Glass) conducting glass. The film thickness was varied from 2.6 to 5.6 μm by the number of screen-printing cycles. The screen-printing paste was composed of ~20 nm diameter anatase particles that gave a mesoporous layer with ~32 nm pores. To render high PCE, a ~5-μm scattering layer (400 nm diameter, Catalysts & Chemicals Ind. Co. Ltd. (CCIC), HPW-400) was deposited on the transparent layer. The TiO 2 electrodes were immersed into a 0.1-mM solution of Y123 with 5 mM 3α,7α-dihydroxy-5β-cholic acid (chenodeoxycholic acid) in 4- tert -butanol/acetonitrile mixture (1:1 v/v) and kept for 15 h at room temperature. The electrolyte consists of 0.22 M [Co(bpy-pz) 2 ] 2+ , 0.05 M [Co(bpy-pz) 2 ] 3+ , 0.1 M LiClO 4 , and 0.2 M 4- tert -butylpyridine in acetonitrile. The I 3 − /I − electrolyte, in the same molar ratio of components as the cobalt, in addition, has 0.17 M 1,3-dimethylimidazolium iodide, 0.05 M iodine, 0.1 M LiI, and 0.2 M 4- tert -butylpyridine in 15/85 (v/v) mixture of valeronitrile and acetonitrile. The dye-adsorbed TiO 2 electrode and thermally platinized counter electrode or PProDOT counter electrode on FTO (TEC 15 ohms per sq, Pilkington) were assembled into a sealed sandwich type cell with a gap of a hot-melt ionomer film, Surlyn (25 μm, Du-Pont). A self-adhesive, anti-reflecting, ultraviolet cutoff film (λ<380 nm, ARKTOP, ASAHI Glass) was attached to the top of active area to decrease light reflection loss. For photovoltaic measurements of the DSCs, the irradiation source was a 450 W xenon light source (Osram XBO 450) with a filter (Schott 113), whose power was regulated to the AM 1.5G solar standard by using a reference Si photodiode equipped with a colour-matched filter (KG-3, Schott) to reduce the mismatch in the region of 350–750 nm between the simulated light and AM 1.5G to less than 4%. The measurement-settling time between applying a voltage and measuring a current for the J–V characterization of DSCs was fixed to 80 ms. The incident photon to collected electron conversion efficiency (IPCE) measurement was plotted as function of wavelength by using the light from a 300-W xenon lamp (ILC Technology), which was focused through a Gemini-180 double monochromator (Jobin Yvon) onto the photovoltaic cell under test. A computer-controlled monochromator was incremented through the spectral range (300–900 nm) to generate a photocurrent action spectrum with a sampling interval of 10 nm and a current sampling time of 4 s. To reduce scattered light from the edge of the glass electrodes of the dyed TiO 2 layer, a light-shading mask was used on the DSCs, so the active area of DSCs was fixed to 0.2 cm 2 . Impedance spectroscopy EIS was performed by an Autolab PGSTAT30 (EcoChemie B.V) in a frequency range between 1 MHz and 0.1 Hz for forward-bias potentials between 0 to 1.1 V (with a 10-mV sinusoidal AC perturbation) in 50 mV steps. The resulting impedance spectra were analysed with ZView software (Scribner Associate) on the basis of the two-channel transmission line model [37] . The results of the EIS are plotted against IR-drop corrected potential. Laser spectroscopy Dye-loaded, 2.8-μm-thick transparent nanocrystalline TiO 2 films were photoexcited by short light pulses (5 ns full-width at half-maximum duration) generated by an optical parametric oscillator pumped by a frequency-tripled Q-switched Nd:YAG laser (Ekspla NT-340). The excitation wavelength was tuned at λ =580 nm. The excitation laser beam was attenuated by grey filters and expanded by plano-concave lens so as to reduce the light pulse fluence on the sample below 20 μJ cm −2 . These conditions ensure that, at most, one electron is injected per TiO 2 particle at a time. The probe light from a Xe arc lamp was passed through filters, various optical elements, the sample, and a second grating monochromator, before being detected by a fast photomultiplier tube and recorded by a digital oscilloscope. The transient probe signal measured at λ =715 nm corresponds to the time evolution of the absorbance of the oxidized state of the dye (S + ) as deduced from previously recorded transient absorption spectra. The transient decay observed corresponds to the lifetime of S + in the presence or absence of a redox electrolyte. The samples measured without any redox species were covered with an acetonitrile film. Traces used to calculate the kinetics of S + decay were typically averaged over 3,000 consecutive laser shots. How to cite this article: Yum, J.-H. et al . A cobalt complex redox shuttle for dye-sensitized solar cells with high open-circuit potentials. Nat. Commun. 3:631 doi: 10.1038/ncomms1655 (2012).